Single-cell and subcellular pharmacokinetic imaging allows insight into drug actionin vivo Pharmacokinetic analysis at the organ level provides insight into how drugs distribute throughout the body, but cannot explain how drugs work at the cellular level. Here we demonstrate in vivo single-cell pharmacokinetic imaging of PARP-1 inhibitors and model drug behaviour under varying conditions. We visualize intracellular kinetics of the PARP-1 inhibitor distribution in real time, showing that PARP-1 inhibitors reach their cellular target compartment, the nucleus, within minutes in vivo both in cancer and normal cells in various cancer models. We also use these data to validate predictive finite element modelling. Our theoretical and experimental data indicate that tumour cells are exposed to sufficiently high PARP-1 inhibitor concentrations in vivo and suggest that drug inefficiency is likely related to proteomic heterogeneity or insensitivity of cancer cells to DNA-repair inhibition. This suggests that single-cell pharmacokinetic imaging and derived modelling improve our understanding of drug action at single-cell resolution in vivo . Drug actions on the human body depend strongly on pharmacokinetics (PK), which describe drug absorption, distribution and elimination. Current PK models typically assume that drugs partition between organ compartments, interacting by mass action transport. Some models include limited molecular and cellular detail, such as receptor occupancy, but in general models tend to focus on coarse-grain processes, such as a single rate constant for tumour cell growth or cell death. Despite such simplifications, these models have nevertheless had a critical role in the latter stages of drug development and in clinical studies, including information on population PKs [1] . Their coarse-grained nature typically precludes their use to understand drug responses in terms of specific signalling pathways or cellular decision-making, and data from PK models are not easily correlated with ‘omic’ data. Perhaps more importantly, existing models tend to neglect heterogeneity in single cell behaviour. This can be especially problematic for cancer drugs, as tumours exhibit high cell-to-cell variability in both epigenetic [2] and genetic [3] properties. Such heterogeneity can arise from different sources [4] , including mutations, varying protein levels due to stochastic gene expression [2] , cell cycle status, tumour position, the degree of interaction with neighbouring cells, as well as different stem cell characteristics [5] , [6] , [7] . Moreover, drug effects can also vary owing to fluctuations in target molecules [3] , resistance mechanisms [8] , interconnected cell signalling networks within cancer cells [9] and influences of the local tumour microenvironmental (such as oxygen concentration [10] , soluble signalling molecules, cell adhesion-mediated interactions [11] and external stimuli). Given this high degree of cellular heterogeneity in tumours, PK measurements and models that account for single-cell dynamics might be more predictive than classic bulk-tissue approaches. Yet, surprisingly little data exist on how specific drugs actually distribute and work in vivo . As autoradiography of radiolabelled drugs cannot achieve the subcellular spatial and temporal resolution possible with fluorescence techniques, studying small-molecule drug distribution remains difficult [12] , [13] , [14] . Recent advances in high-resolution subcellular in vivo imaging methods have enabled more detailed analyses of single cells and, as such, are now being increasingly used to understand how cancer cells behave in in vivo environments [15] , [16] , [17] , [18] . Furthermore, parallel advances in synthetic methods have facilitated the development of small-molecule fluorescent drugs with similar affinity and PKs to their therapeutic counterparts [19] , [20] . One approach to measuring and modelling drug kinetics would thus be to use optimally labelled drugs for high-resolution in vivo fluorescence imaging ( Fig. 1 and Supplementary Fig. S1 ). Single-cell in vivo PK imaging could then be used to shed new light on several aspects of drug development in that it would allow measurement of intratumor heterogeneity, analysis of drugs that target the tumour microenvironment, mechanistic-driven optimization of drug doses (after appropriate adjustment for drug-specific properties), comparison of different closely related compounds, correlation of drug concentrations to effector function, extrapolation of simulations to humans, as well as the performance of detailed failure analyses. 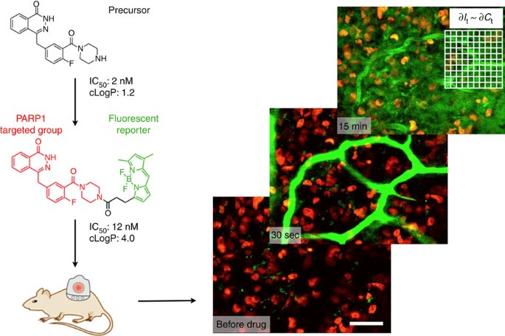Figure 1: High spatial and temporal resolution microscopy using companion imaging drugs. Precursor compounds are conjugated with cell permeable, small fluorophores to generate therapeutically active fluorescent companion imaging drugs (seeSupplementary Fig. S1for structure of parent drug and how piperazine substitutions are tolerated48). Using a window chamber model,in vivomicroscopy enabled the detection of drugs (green) with subcellular resolution and frame rates of several seconds. Scale bar, 50 μm in an MDA-MB-231 breast cancer cell line expressing a fluorescent H2B protein in the nucleus (red). Figure 1: High spatial and temporal resolution microscopy using companion imaging drugs. Precursor compounds are conjugated with cell permeable, small fluorophores to generate therapeutically active fluorescent companion imaging drugs (see Supplementary Fig. S1 for structure of parent drug and how piperazine substitutions are tolerated [48] ). Using a window chamber model, in vivo microscopy enabled the detection of drugs (green) with subcellular resolution and frame rates of several seconds. Scale bar, 50 μm in an MDA-MB-231 breast cancer cell line expressing a fluorescent H2B protein in the nucleus (red). Full size image Here we develop new imaging and analysing tools, validate them and then undertake a model study using in vivo imaging to analyse drug distribution in murine cancer models. Specifically, we develop high-resolution, temporal in vivo imaging of single cells in tumours to measure drug distribution, synthesize a fluorescent derivative of a PARP inhibitor (PARPi) that retained activity and utilize a quantitative framework to extract and extrapolate single cell data to be used in predictive models. We chose PARPi as an emerging area of solid tumour pharmacology, with an exciting rationale of synthetic lethality [21] , potent and specific compounds, and unexpectedly low success in the clinic for unexplained reasons [22] , [23] . We believe that this approach of single-cell PK imaging (SCPKI; Supplementary Fig. S1 ) could prove valuable in understanding drug action for different drugs and diseases. Development of imaging technique and PARPi characterization During SCPKI, serial images and stacks were obtained in representative areas of the tumour ( Fig. 1 ). Typically, 20–60 × objectives were used to discern intracellular detail of ~50–300 cells per field, whereas multiple fields were sampled in z, using objective and stage automation. Several features of the set-up were further optimized for SCPKI. Assuming that the position of single cells changes over several hours of observation, we applied robust immobilization and cell-tracking techniques in addition to acquiring image stacks. Time series were initiated before intravenous injection, allowing dynamic scanning during partition of drug from circulation into the tumour. This allowed capture of critical early phases of drug distribution. Anaesthesia was monitored and adjusted to maintain stable vital signs over a 4- to 6-h imaging session. Intravenous fluids were supplied, and animals were warmed appropriately to avoid hypothermia [18] . 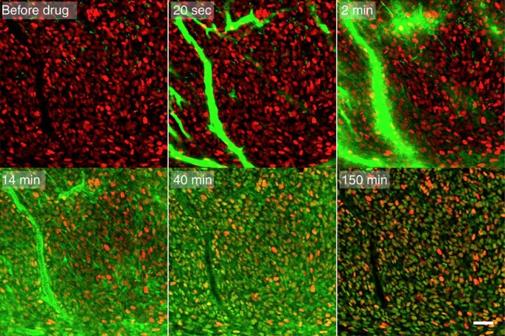Figure 2: Real-timein vivodrug distribution of a PARP inhibitor. Following bolus intravenous administration, the drug (green) perfused the functional tumour vasculature within seconds and extravasated within minutes (top row). The drug initially distributed non-specifically within H2B-RFP (red)-expressing cells (primarily within the endoplasmic reticulum, as determined byin vitrocell imaging;Supplementary Fig. S4, HT-1080 cell line shown). Rapid target binding (within minutes) combined with clearance of non-specific membrane labelling increased the specificity of target versus non-target uptake within an hour. Specific nuclear PARP targeting was observed (bottom row) and this was maintained for several hours. SeeSupplementary Movie S1for dynamic imaging. Scale bar, 50 μm. Figure 2 and Supplementary Movie S1 shows a representative example of a raw data set following bolus tail vein injection of the fluorescently tagged PARPi ( Fig. 1 and Supplementary Fig. S2 ). The drug filled the functional tumour vasculature within seconds after injection and extravasated within minutes, distributing non-specifically to cells, and then washing out to reveal target binding in the nucleus of the vast majority of cells ( Fig. 3 ). Figure 2: Real-time in vivo drug distribution of a PARP inhibitor. Following bolus intravenous administration, the drug (green) perfused the functional tumour vasculature within seconds and extravasated within minutes (top row). The drug initially distributed non-specifically within H2B-RFP (red)-expressing cells (primarily within the endoplasmic reticulum, as determined by in vitro cell imaging; Supplementary Fig. S4 , HT-1080 cell line shown). Rapid target binding (within minutes) combined with clearance of non-specific membrane labelling increased the specificity of target versus non-target uptake within an hour. Specific nuclear PARP targeting was observed (bottom row) and this was maintained for several hours. See Supplementary Movie S1 for dynamic imaging. Scale bar, 50 μm. 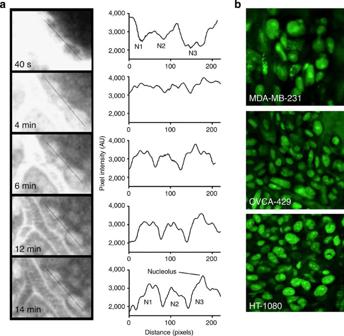Figure 3: Subcellular spatial resolution of drug distribution. (a) A line profile through three cells adjacent to a tumour vessel shows perinuclear signal within seconds after injection (PARPi fluorescence shown in grey scale). Accumulation in the nucleus and diffusion of free drug deeper into the tumour results in nuclear-specific staining with the contrast increasing over time. A high signal in the nucleolus can be observed in these HT-1080 cells with similar staining patterns in multiple cell lines. (b) High-resolution images of intracellular (primarily nuclear) drug distribution in three different cancer modelsin vivo. PARPi fluorescence shown in green. Full size image Figure 3: Subcellular spatial resolution of drug distribution. ( a ) A line profile through three cells adjacent to a tumour vessel shows perinuclear signal within seconds after injection (PARPi fluorescence shown in grey scale). Accumulation in the nucleus and diffusion of free drug deeper into the tumour results in nuclear-specific staining with the contrast increasing over time. A high signal in the nucleolus can be observed in these HT-1080 cells with similar staining patterns in multiple cell lines. ( b ) High-resolution images of intracellular (primarily nuclear) drug distribution in three different cancer models in vivo . PARPi fluorescence shown in green. Full size image Supplementary Figure S2 summarizes the synthesis and physicochemical characterization of the PARP-imaging agent, based on covalent modification of the olaparib (AZD2281) scaffold with a boron-dipyrromethene (BODIPY) N -hydroxysuccinimide ester. The fluorescent companion drug (emission maximum: 525 nm) has a molecular weight of 640 Da and displays excellent characteristics as a targeted fluorescent reporter group, as its affinity is not greatly perturbed by the attachment of a fluorescent BODIPY-FL reporter. The half-maximal inhibitory concentration (IC 50 ) was determined as 12.2±1.1 nM ( Supplementary Fig. S3 ), which is higher than the parent drug, but still in the low nanomolar range. Although olaparib has been shown to affect multiple members of the PARP family [24] , only PARP-1 had significant expression and drug affinity in the model systems used. PARP-2 was absent and the affinity for PARP-3 was too low for a therapeutic effect in vivo ( Supplementary Fig. S4 ). The fluorescent compound freely permeates into cells and colocalizes with PARP immunostaining ( Supplementary Figs S4 and S5 ) at the single-cell level as well as in different cell lines tested, including breast cancer (MDA MB231), ovarian cancer (OVCA429) and others (HT1080, A431). Supplementary Fig. S6 summarizes the cellular kinetics of target accumulation in breast cancer cells in culture where unbound compound was removed from the cells within minutes, resulting in relatively fast intracellular kinetics. To directly correlate the fluorescence signal with drug concentrations, we used phantom data ( Supplementary Fig. S3 ), which we validated in vivo using a built-in calibration (injected dose in vessels; Fig. 2 and Supplementary Fig. S7 ). Together, these data show that drug concentrations can be estimated inside cells and followed over time; we observed little, if any, bleaching over typical observation periods and settings. At the whole-body level, the imaging drug had a weighted blood half-life of 18 min (77% redistribution with a 5-min half-life and a 23% clearance phase of 60 min; Supplementary Fig. S7 ); competitive inhibition of target binding could be achieved through administration of cold drug ( Supplementary Fig. S3D ). Single-cell distribution of PAPRi measured in vivo To determine drug concentrations in vivo in individual tumour cells, we segmented cells in two-dimensional images based on nuclear expression of the fluorescent protein H2B-apple and used a semi-automated algorithm to define associated cell mass ( Fig. 4 ). Fluorescence per cell was then displayed for each individual cell as well as for populations of cells over time. A representative image is shown in Fig. 4 along with the s.d. between cells as a function of time. Of note, the s.d. was large immediately after drug administration owing to variability in delivery (primarily in proximity to functional blood vessels). Within an hour, however, the heterogeneity decreased and continued to decrease over time, as the drug diffusion reduced the gradients within the tissue. Three hours after intravenous administration, the cellular drug concentration was 1.2±0.2 μM, regardless of intratumoral position. At this time point, >99% of the tumour cells are predicted to have therapeutic drug levels based on extrapolation of the dose and measured variability in drug concentrations observed in different tumour cell beds. These cell-population kinetics thus allowed the study of drug distribution to cells within different tumoral regions (that is, to cells adjacent to vessels, to cells as a function of vascular distance or in relatively avascular regions). It also enabled measurement of the fraction of cells receiving no drug or subtherapeutic drug levels (see below). 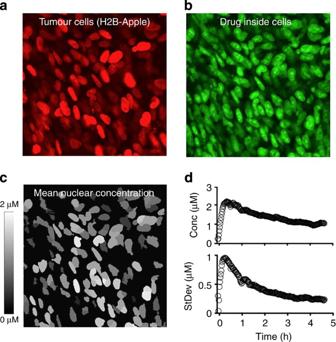Figure 4: Cell population drug kinetics. (a) H2B-Apple red fluorescent protein was used to identify the nuclei of individual cancer cellsin vivo(model HT-1080 cell line shown). (b) The drug (green) accumulates inside cells, specifically in the nuclei. (c) To measure the average drug concentration inside each cell, nuclei were segmented (based ona) and outlines were overlaid with the companion imaging drug to yield a mean nuclear concentration (c). Note that the average cellular drug concentration in thisin vivoexample is 1.2 μM. Although virtually all cancer cells accumulated the drug (>99%), there was still some cell-to-cell variability. (d) The average concentration rapidly increases following a bolus dose followed by a slow decay (top). Analysing the s.d. of 250 cells over time showed the highest deviation at early time points decreasing to a much lower level as the diffusive gradients dissipated (bottom). Figure 4: Cell population drug kinetics. ( a ) H2B-Apple red fluorescent protein was used to identify the nuclei of individual cancer cells in vivo (model HT-1080 cell line shown). ( b ) The drug (green) accumulates inside cells, specifically in the nuclei. ( c ) To measure the average drug concentration inside each cell, nuclei were segmented (based on a ) and outlines were overlaid with the companion imaging drug to yield a mean nuclear concentration ( c ). Note that the average cellular drug concentration in this in vivo example is 1.2 μM. Although virtually all cancer cells accumulated the drug (>99%), there was still some cell-to-cell variability. ( d ) The average concentration rapidly increases following a bolus dose followed by a slow decay (top). Analysing the s.d. of 250 cells over time showed the highest deviation at early time points decreasing to a much lower level as the diffusive gradients dissipated (bottom). Full size image To better understand the temporal changes in drug concentrations in individual cells, we performed kinetic measurements in vivo over 4 h ( Fig. 5 ). Interestingly, we observed some variation in maximum uptake, but much less variation in cellular drug concentration at later time points. As shown in the representative kinetograms in Fig. 5 , the average drug concentration within a given cell was 1.2 μM after 4 h. We subsequently analysed the distribution of drug at early (20 min) and late (90 min) time points in populations of cells. The log normal distributions are plotted for representative mice and tumour types ( Fig. 5 ). At early time points, average cellular drug concentration was primarily related to vessel proximity, whereas at later time points it appeared to be governed by stochastic distribution. Although cell movement was too great to isolate clonal populations within the tumour (with many cells migrating at 10–20 μm h −1 ), there was no discernible structure to the distribution. Although uptake of this probe correlates with the PARP-1 expression in cell culture [25] , where there are no transport limitations or tumour microenvironmental effects, no correlation existed when digested tumours were analysed by flow cytometry (data not shown), although loss of drug during preparation could not be completely ruled out. In some of these experiments, we performed repeated bolus injections to determine whether drug concentrations within cells were additive and related in magnitude. The signal increase after the second injection was smaller than that after the first injection, likely because of a saturation phenomenon. The heterogeneity between cells, although unexpected, could be the result of variability in target expression, the cell cycle phase (for example, DNA content), differences in stochastic gene expression, nuclear volume and/or genetic mutations. Variability in the competitive NAD concentration in the cell could also affect the binding, although the in vitro affinity was measured in the presence of NAD with the current probe. This method could be adopted to measure the concentration of competitive inhibitors, such as NAD, in vivo . 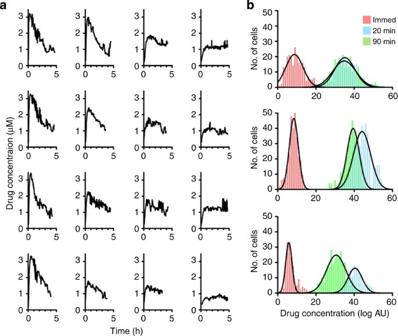Figure 5: Single-cell drug kinetics. Individual cell profiles can be tracked by temporal single cell imagingin vivo. (a) Drug concentrations inside cancer cells were plotted as a function of time following intravenous administration and according to their proximity to microvessels. Profiles in the left column are from representative single cancer cells adjacent to microvessels, profiles in the right column are from cells ~200 μm away from the nearest vessel, and the columns in the middle are from cells at intermediate distances. Note that the intracellular drug concentration in cells is similar at 4 h after administration. (b) A histogram of the log-normal population kinetics over time in different cancer cell types. Top: breast cancer (MDA-MB-231), middle: ovarian cancer (OVCA-429) and bottom: fibrosarcoma (HT-1080). Differences in heterogeneity primarily correspond to changes in vascular density. Figure 5: Single-cell drug kinetics. Individual cell profiles can be tracked by temporal single cell imaging in vivo . ( a ) Drug concentrations inside cancer cells were plotted as a function of time following intravenous administration and according to their proximity to microvessels. Profiles in the left column are from representative single cancer cells adjacent to microvessels, profiles in the right column are from cells ~200 μm away from the nearest vessel, and the columns in the middle are from cells at intermediate distances. Note that the intracellular drug concentration in cells is similar at 4 h after administration. ( b ) A histogram of the log-normal population kinetics over time in different cancer cell types. Top: breast cancer (MDA-MB-231), middle: ovarian cancer (OVCA-429) and bottom: fibrosarcoma (HT-1080). Differences in heterogeneity primarily correspond to changes in vascular density. Full size image The above methods allowed us to address another important question—what is the drug exposure in non-cancerous cells in the tumour? Tumours typically comprise a mixture of cancer cells together with varying amounts of stroma and infiltrating leukocytes. In our models, tumour cells were found to be the predominant cell type (breast cancer model: ~80% tumour cells, ~20% host cells). Yet, in other models such as human cancers and murine K-ras models [26] , tumour-associated macrophages (TAMs) can be much more prevalent. We found that PARPi distributed non-discriminately to all cells, including endothelial and host cells, with similar kinetics as for cancer cells. However, the absolute magnitude of cellular accumulation was found to differ, with the highest concentrations accumulating in cancer cells ( Fig. 6 ). This may be, in part, because of the fact that host cells have lower levels of PARP1 or simply because they are smaller cells. 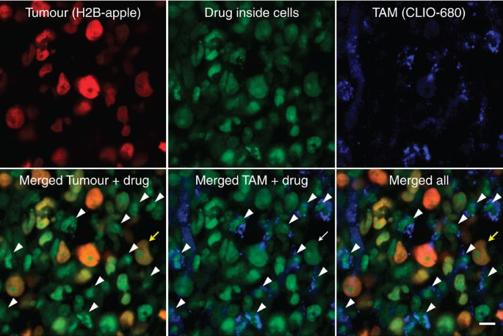Figure 6: Mapping drug distribution to host cells. Within a tumour, cancer cells were visualized through expression of H2B-Apple (580 nm, red) and TAMs were visualized by a fluorescent nanoparticle (680 nm, blue) internalized into endosomes. The PARPi distribution to cells was visualized at 525 nm (green). The PARPi was seen to accumulate in cancer cells (yellow arrow, HT-1080 cell line), but also in TAMs (as indicated by the white arrowheads). TAM nuclei lack the H2B-apple and are surrounded by CLIO signal. Scale bar, 10 μm. Figure 6: Mapping drug distribution to host cells. Within a tumour, cancer cells were visualized through expression of H2B-Apple (580 nm, red) and TAMs were visualized by a fluorescent nanoparticle (680 nm, blue) internalized into endosomes. The PARPi distribution to cells was visualized at 525 nm (green). The PARPi was seen to accumulate in cancer cells (yellow arrow, HT-1080 cell line), but also in TAMs (as indicated by the white arrowheads). TAM nuclei lack the H2B-apple and are surrounded by CLIO signal. Scale bar, 10 μm. Full size image Finite element modelling of PARPi distribution Although the above data was informative in its own right, we hypothesized that quantitative image analysis and modelling could be used to extrapolate findings and investigate biological variables (for example, vascularity, tumour types, mitotic rates), which would otherwise require extensive biological experiments or simply not be practical (for example, extrapolation to humans). A major obstacle in developing these refined models has been the lack of experimental data to validate any such model. We developed a two-compartment subcellular (nuclear and cytoplasmic), non-linear, partial differential equation model ( Fig. 7 ) to simulate and display major trends in tissue distribution, and directly compared the modelled data with the real experimentally obtained data ( Fig. 8 ). The employed model did not represent single cells, but had unique advantages, including the ability to evaluate and refine the model based on experimental imaging data, and rapidly model in silico the distribution of any arbitrary vascular framework. This approach may be used to account for the stochastic nature of tumour vasculature [27] . Once the blood clearance is known, simulation results can be adapted to different delivery routes (that is, infusion, intraperitoneal, subcutaneous) and species, including humans; insight is also provided on how specific drug properties (permeability, non-specific uptake, diffusion) affect intratumoral distribution. Interestingly, the permeability of the PARPi did not differ statistically between a window chamber ( Figs 2 and 6 ), orthotopic mammary fat pad tumour ( Supplementary Figs S8 and S9 ), or normal vasculature of the ear ( Supplementary Fig. S10 ). Although it is known that macromolecular permeability varies depending on tumour location [28] , these results help validate the previous prediction that small-molecule drugs are not limited by permeability [29] . 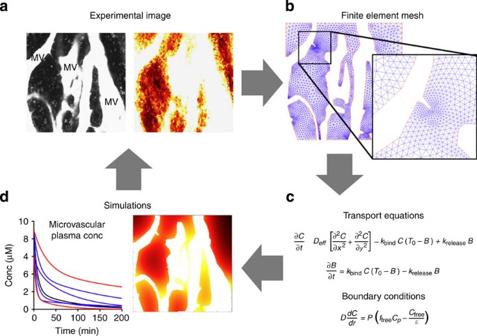Figure 7: Simulation development and validation. Small molecule drugs distribute to cancer cells from functional tumour microvasculature. (a) In the model system, tortuous microvessels were mapped using lectins or vascular probes (top left). (b) A finite element mesh was generated around the vessel maps. (c) Transport equations and boundary conditions were applied to the simulation. (d) Simulation results for time and spatially varying drug concentrations could then be compared with the intravital imaging time series (a) for validation or improvement. These simulations could likewise be extrapolated to different species and used to study the effects of other specific variables. SeeSupplementary Fig. S6for specific numerical parameters. Figure 7: Simulation development and validation. Small molecule drugs distribute to cancer cells from functional tumour microvasculature. ( a ) In the model system, tortuous microvessels were mapped using lectins or vascular probes (top left). ( b ) A finite element mesh was generated around the vessel maps. ( c ) Transport equations and boundary conditions were applied to the simulation. ( d ) Simulation results for time and spatially varying drug concentrations could then be compared with the intravital imaging time series ( a ) for validation or improvement. These simulations could likewise be extrapolated to different species and used to study the effects of other specific variables. See Supplementary Fig. S6 for specific numerical parameters. 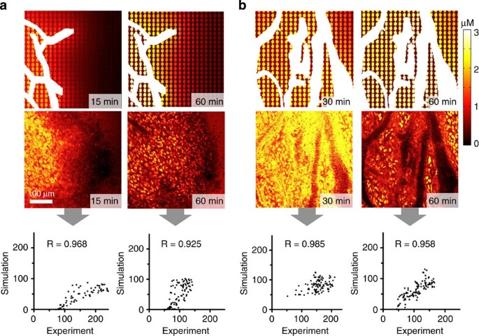Figure 8: Predictive models of PARPi distribution. Vessel heterogeneity can be a major determinant of drug distribution particularly early after administration. In these examples (using HT-1080 xenografts with wide variation in vascular density within the same tumour) drug gradients are modelled as a function of distance from microvessels (white); each oval shape represents a model cell. (a) A poorly vascularized region shows a large gradient at early times (15 min; left) for both the simulation (top) and the corresponding intravital image (bottom). By 1 h (right), the gradient is significantly reduced and intracellular drug concentrations reach ~1 μM levels. The large Mander correlation coefficient validates the model predictions based onin vitroexperimental measurements and systemic clearance. (b) High vessel density reduces the spatial gradients, and the cellular accumulation reaches 2-3 μM following administration of the imaging dose. These types of simulations can be used to determine the impact of changing the drug physiochemical properties on distribution for both therapeutics and imaging agents. SeeSupplementary Fig. S8for additional modelling including human extrapolation. Full size image Figure 8: Predictive models of PARPi distribution. Vessel heterogeneity can be a major determinant of drug distribution particularly early after administration. In these examples (using HT-1080 xenografts with wide variation in vascular density within the same tumour) drug gradients are modelled as a function of distance from microvessels (white); each oval shape represents a model cell. ( a ) A poorly vascularized region shows a large gradient at early times (15 min; left) for both the simulation (top) and the corresponding intravital image (bottom). By 1 h (right), the gradient is significantly reduced and intracellular drug concentrations reach ~1 μM levels. The large Mander correlation coefficient validates the model predictions based on in vitro experimental measurements and systemic clearance. ( b ) High vessel density reduces the spatial gradients, and the cellular accumulation reaches 2-3 μM following administration of the imaging dose. These types of simulations can be used to determine the impact of changing the drug physiochemical properties on distribution for both therapeutics and imaging agents. See Supplementary Fig. S8 for additional modelling including human extrapolation. Full size image We first validated the model by directly comparing outputs with experimentally acquired data. We initially focused on vascular density ( Fig. 8 ) and later expanded the predictions to other variables, such as intermittent flow ( Supplementary Fig. S11A ) and human dosing ( Supplementary Fig. S11B ). Experimental data showed that poorly vascularized regions showed a strong spatial gradient at 15 min, which started to dissipate after 1 h ( Fig. 8a ). The non-specific tumoral distribution at early time points cleared to reveal nuclear specific staining at later time points. Interestingly, there was remarkably good agreement between purely model data and real experimental data. Figure 8 shows the overall agreement and the calculated Mander’s correlation coefficients for individual data sets. It is important to note that the simulations only use the vascular architecture for experimental input; the curves are not fit to the microscopy data. Rather, independent in vitro experiments are used to estimate the driving forces for transient drug distribution ( Supplementary Table S1 ) to allow true predictions of drug uptake in vivo . This also allows data from in vitro experiments on non-fluorescent drug variants to be utilized in the simulations. For regions with much higher vascular density ( Fig. 8a ), increased delivery resulted in higher drug concentrations and a more homogeneous distribution. The model was subsequently used to predict the distribution profile around vessels with intermittent blood flow [30] . Although intermittent blood flow caused transient changes in drug distribution (in addition to a prediction of acute hypoxia) at early time points, the diffusion from surrounding vessels and the time-averaged delivery of the drug by the vessel of interest resulted in a low impact at later time points ( Supplementary Fig. S11A ). Perhaps, one of the most useful aspects of modelling is the ability to extend the data to other species (human) by scaling the plasma clearance rates and adjusting drug-specific parameters (molecular weight, oral bioavailability, drug transporter affinity and so on). As an example, the slower absorption and clearance of drugs after oral delivery in humans [31] resulted in the prediction of a lower drug gradient for this compound in the clinic. This represents one of the most important strengths of developing predictive simulations—the ability to provide insight into situations that are difficult to measure experimentally (for example, the temporal tissue, and cellular and subcellular distribution of drugs in human tumours). These models can then be used for hypothesis-driven research, which will either validate or refute the predictions in human tumours when future improvements in technology allow such measurements. Supplementary Fig. S11B shows the maximum predicted gradient following orally administered drug (b.i.d.) at steady state compared with the concentration before the next dose in a poorly vascularized region. The oral availability was assumed the same as the clinical drug, although the simulation allows arbitrary adjustment of this parameter to investigate the impact of bioavailability on distribution. The relatively quick absorption after oral dosing (<2 h) resulted in gradients within the tissue for regions that were poorly vascularized. A small gradient in the opposite direction was found at time points before dosing, as the drug slowly washed out from the tissue. Notably, cells adjacent to the vessels had larger temporal changes in concentration, whereas those further away were buffered from these changes by a depot effect. Overall, these gradients were much lower than in mouse models, owing to slower systemic absorption and clearance in humans. Our results indicate that at current clinical doses, virtually all cells in a human tumour (>99%, including cancer and non-cancer cells) should attain therapeutic drug concentrations and maintain them over the entire treatment period with this compound. Using the model, generic scenarios in which subtherapeutic concentrations might occur in clinical settings can be predicted and differentiated, including the following scenarios with the potential to cause drug failure: (1) low systemic doses (for example, as a result of poor oral availability); (2) rapid clearance or metabolism where trough plasma concentrations are low enough to wash out the drug between doses; (3) non-continuous dosing where the drug fails to reach distant cells before therapy is discontinued (this is more likely when there is significant drug binding to tissue, for example, with drugs targeting DNA, microtubules, or high target density molecules); (4) local metabolism within the tumour tissue; (5) local active transport out of the target region (for example, when there is high p-glycoprotein expression); (6) changes in effective therapeutic concentrations such as might occur when there is increased expression of competitors (for example, ATP for kinase inhibitors); or (7) mutations in the binding pocket reducing drug affinity. Our study demonstrates that robust high-resolution profiles of drug distribution over time in single cells in model tumours can be obtained, and that by examining multiple cells from the same mouse tumour, inferences about global effects can be made. Moreover, quantitative data can be either modelled to predict cumulative drug effects or extrapolated to human settings to provide insights into drug action previously undetectable by other methods. The findings with PARPi in the present study demonstrate the drug’s ubiquitous distribution to virtually all cells in a tumour, including non-cancerous cells, rapid permeation to the nucleus and sustained binding to target in the nucleus. Given the lower molecular weight and reduced lipophilicity (logP) of the clinical compound, olaparib is predicted to distribute slightly faster than the fluorescent derivative analysed here, leading to conservative estimates with these predictions. These observations suggest that clinically observed failures with olaparib are less likely attributable to delivery failures. Rather, our findings are more consistent with recent mechanistic studies [32] , [33] , which have all indicated that BRCA (but not triple negative breast cancer) mutations are required for drug efficacy. There are a number of different global models describing drug distribution and response; these include population PK models [1] , physiologically based PK models [34] , [35] , [36] , empirical PK/pharmacodynamic (PD) models and mechanistic (for example, receptor binding) PK/PD models, among others [37] . Although these models have been developed to incorporate delivery limitations or more complex PD measures, there is currently no method that incorporates the known cell-to-cell variability in cancer phenotypes, the multivariate cell decision inputs, the heterogeneous nature of drug delivery and the variability of cellular responses into a comprehensive framework. To reconcile the gap between these global models and molecular pathways at the cellular level [38] , [39] , we have been working on developing intravital imaging techniques that are capable of providing insight into drug dose–response relationships at the single cell level. Supplementary Fig. S1 summarizes our approach and compares it with global measurements and related modelling methods. A central aspect of the quantitative measurements obtained using the described technique is the development and use of companion imaging drugs that display similar efficacy and in vivo behaviours to the parent drug [19] . The magnitude and evolution of drug gradients can thus be measured and subsequently modelled using finite element-based simulations. These results can also be extrapolated to other species based on plasma concentration time profiles. We examined only two cancer types in depth; both exhibited ubiquitous distribution of the fluorescent PARPi. Using image quantification and numerical simulations, we found that intracellular drug concentrations will reach sufficiently high levels (above the IC 50 ) in most breast and ovarian cancer cells lines, and exceeding that in BRCA−/− models by an order of magnitude (Katy S. Yang, unpublished data) with current preclinical dosing levels. Using a model-based extrapolation of clinical physiological and drug parameters to humans, we infer that the qualified failure of PARPi in recent trials are likely failures of efficacy rather than failures of delivery [22] . Measuring drug concentrations by intravital imaging at the single-cell level could be further expanded to other drug classes (for example, siRNA, antibodies, nanocarriers), other engineered cell and tumour models. First, the experimental window chamber set-up enables rapid analysis and screening of different cancer types; indeed, this set-up is currently being used to evaluate several drugs of interest. Of note, the permeability of this small-molecule drug was not statistically different in the window chamber, an orthotopic model, or the normal vasculature of the ear ( Supplementary Figs S8 and S10 ) as also predicted by transport models [29] , enabling the use of the window chamber for most experiments with this class of agent. Second, the method allows drug response to be tested in the presence of key mutations (for example, the BRCA status, oncogene mutations). Third, it is possible to conduct mixing experiments where mosaic cells from different backgrounds (encoded by different fluorescent proteins) are studied in parallel to determine differences in drug effects in vivo (for example, using FUCCI reporters to detect cell cycle effects [40] , using resistant and sensitive cell lines encoded by different fluorescent proteins, or using clonal cell populations [41] ). Fourth, through the use of reporter genes it is possible to link kinetic data to the PD data. Although in the present study we used morphological nuclear features as a predictor of apoptosis [42] , fluorescent reporter genes such as 53BP1-XFP [43] , Ki67-XFP [44] or p21-XFP [45] could also be used. Fifth, the model enables in vivo synergy and distribution to be determined by using combinations of differently tagged drugs. BODIPY fluorochromes in particular have a relatively small footprint and can be synthesized in a variety of excitation/emission ranges [46] . Finally, because of advances in optics and objectives [47] , and through the use of newer immobilization and gating techniques, it has recently become possible to study drug distribution directly in orthotopic cancers without the use of window chambers. Together, these advances will enable the field of single-cell PK and PD imaging/modelling to directly connect information on cancer cell signalling networks to therapeutic efficacy. Synthesis Synthesis of the companion imaging drug AZD2281-BODIPY FL was carried out as described in Supplementary Fig. S2A . Specifically, we reacted a solution of BODIPY-FL succinimidyl ester (5.0 mg, 12.8 μmol; Invitrogen, Carlsbad, CA, USA) in acetonitrile (250 μl), with a solution of 4.7 mg (12.8 μmol, dissolved in 250 μl acetonitrile) of 4-4-fluoro-3-(piperazine-1-carbonyl)phenylmethyl]-2 H -phthalazin-1-one [48] in the presence triethylamine (4.6 μl, 64.2 μmol). The two components reacted within 4 h at room temperature. The product AZD2281-BODIPY FL was then isolated using standard HPLC techniques performed on a Waters’ (Milford, MA) liquid chromatography–mass spectrometry (LC-MS) system and using a Waters’ XTerra C18 5 μm column. The title compound was isolated in 72% yield and its identity confirmed using LC/MS, HPLC, NMR and high-resolution mass spectrometry techniques ( Supplementary Fig. S2B,C ). The compound had a maximum absorbance at 507 nm and a maximum emission at 527 nm ( Supplementary Fig. S2A ). 1 H NMR (600 MHz, dimethyl sulfoxide (DMSO)-d 6 , 297.2 K) δ =12.61 (d, 3 J HH =3.3, 1 H), 8.26 (dd, 3 J HH =7.7, 3.9, 1 H), 8.03–7.93 (m, 1 H), 7.89 (t, 3 J HH =7.6, 1 H), 7.82 (dt, 3 J HH =14.2, 7.5, 1 H), 7.70 (d, 3 J HH =4.1, 1 H), 7.46–7.42 (m, 1 H), 7.37 (t, 3 J HH =6.1, 1 H), 7.24 (t, 3 J HH =8.9, 1 H), 7.09 (t, 3 J HH =4.6, 1 H), 6.42 (dd, 3 J HH =21.4, 4.0, 1 H), 6.30 (d, 3 J HH =4.6, 1 H), 4.33 (d, 3 J HH =3.0, 2 H), 3.68–3.47 (m, 4 H), 3.44–3.35 (m, 2 H), 3.22–3.13 (m, 2 H), 3.11–3.04 (m, 2 H), 2.78 (t, 3 J HH =7.8, 1 H), 2.71 (t, 3 J HH =7.7, 1 H), 2.46 (d, 3 J HH =8.6, 3 H), 2.26 (d, 3 J HH =3.3, 3 H); 13 C NMR (151 MHz, DMSO-d 6 , 297.2 K) δ =169.65, 169.62, 164.07, 164.01, 159.41, 159.11, 157.85, 157.20, 157.15, 155.58, 155.53, 144.87, 144.08, 134.85, 134.42, 133.53, 133.02, 131.81, 131.76, 131.60, 131.58, 129.10, 128.96, 128.93, 127.90, 126.10, 125.49, 125.37, 123.67, 123.61, 123.54, 123.49, 120.27, 117.14, 116.04, 116, 115.90, 115.86, 69.80, 46.56, 46.30, 44.79, 44.37, 41.57, 41.31, 41.26, 40.76, 39.10, 36.46, 31.21, 23.77, 23.74, 14.54, 11.04. 19 F NMR (376 MHz, DMSO- d 6 ) δ =-119.4 (s, 1 F), -142.8 (q, J BF =33 Hz, 2 F); LC-ESI-MS(+) m / z =621.4 [M−F] + , 641.4 [M+H] + , 663.4 [M+Na] + ; LC-ESI-MS(−) m / z =619.3 [M-2 H−F] − , 639.3 [M−H] − ; high-resolution mass spectrometry-ESI [M+H] + m/z calculated. for [C 32 H 33 BF3N 6 O 3 ] + 641.2671, found 641.2688 [M+H] + . Tumour models The human breast cancer cell line MDA-MB-231 was purchased from ATCC (Manassas, VA, USA), and OVCA429 and A2780 cell lines were generously provided by Dr Michael Birrer (Massachusetts General Hospital, Boston, MA, USA). These cell lines were grown in RPMI media supplemented with 10% fetal bovine serum, and 1% penicillin-streptomycin. HT-1080 and A431 cells from ATCC were grown in DMEM supplemented with 10% fetal bovine serum and 1% penicillin–streptomycin. Reporter cell lines Histone 2B-red fluorescent protein (H2B-apple) was used to identify the nuclei of individual cancer cells, as this model has previously been shown to be robust in vivo [42] . pmApple-N1 (Myo1E-pmApple-C1, Addgene, Professor Christien Merrifield [49] ) was cloned by ligating Apple into pmCherry-N1 (Clontech) using Afe I and Bsr G1 restriction enzymes. The pTag-H2B-Apple construct was generated by subcloning mApple from pmApple-N1 into pTag-H2B-BFP (Evrogen) using Age I and Not I. Correct insertion of Apple was confirmed by sequencing the insert in its entirety. For the MDA-MB-231 and OVCA429 cells, H2B-Apple was subcloned from the pTag H2B-Apple vector into the lentiviral vector pLVX (Clontech) containing H2B-FP, using the Bam HI and Not I restriction enzymes. Infectious lentiviral particles were produced in Lenti-X 293 T cells (Clontech) by transfecting cells with pLVX-H2B-Apple using the Xfect transfection reagent (Clontech). The medium (DMEM, 10% Tet-Approved FBS, 100 IU penicillin, 100 μg ml −1 streptomycin and 2 mM L -glutamine) was replaced 6 h after transfection. The lentivirus was collected 72 h after transfection by collecting and filtering supernatant through a 0.45-μm cellulose acetate filter. Lentiviral particles were concentrated using the Lenti-X concentrator (Clontech) and incubated overnight at 4 °C. The supernatant was centrifuged at 1500 g for 45 min at 4 °C. To infect MDA-MB-231 and OVCA429 cells, 5 × 10 4 cells were plated into a 12-well plate and allowed to adhere overnight. Medium was replaced with 1 ml complete growth medium (RPMI, 10% FBS, 100 IU penicillin, 100 μg ml −1 streptomycin, 2 mM L -glutamine) and 50 μl lentivirus was added to the medium along with 4 μg ml −1 polybrene. After overnight incubation, the medium was replaced with fresh growth medium. Fourty-eight hours post-infection, cells were trypsinized and expanded in a 10 cm dish with 3 μg ml −1 puromycin for selection. pTag-H2B-Apple was transfected into HT1080 cells using the X-tremeGENE HP transfection reagent (Roche), followed by selection in 500 μg ml −1 G418. Using a fluorescent microscope, one clone was selected for fluorescence-activated cell sorting, and the brightest 5% of cells were isolated for expansion. Cells were maintained in complete growth medium with 100 μg ml −1 G418. Intravital microscopic imaging All animal experiments were carried out in accordance with guidelines from the Institutional Subcommittee on Research Animal Care. Nude mice (Cox7, Massachusetts General Hospital) were surgically implanted with a dorsal skin window chamber. Approximately 3–4 × 10 6 cells suspended in 1:1 PBS and Matrigel (BD Biosciences, Franklin Lakes, NJ, USA) were implanted under the fascia and allowed to grow for ~2 weeks. When the tumours became vascularized and reached 1–2 mm in size, mice were anaesthetized with 2% isoflurane in 2 l min −1 oxygen on a heated microscope stage and injected via tail vein catheter with either Angiosense-680 (Perkin Elmer, Waltham, MA, USA) or 250 μg of a 500-kDa amino-dextran labelled with Pacific Blue N-Hydroxysuccinimide ester (Invitrogen, Grand Island, NY, USA), according to the manufacturer’s instructions. Vascularized regions of interest in the tumour were identified by the vessel probe and H2B-Apple tumour cell signal; regions with minimal out-of-plane vessels were chosen for imaging. Pre-treatment images were collected and time-lapse imaging initiated before injection of the drug via the tail vein catheter. For experiments in which TAMs were identified, 20–40 mg kg −1 of VT680-labelled dextran nanoparticle (CLIO) was injected 24 h before imaging. A time-lapse imaging series was initiated, and the AZD2281-BODIDY-Fl was injected during image sequence acquisition. The drug was formulated by dissolving 7.5 μl of a 10 mM solution in DMSO along with 30 μl of a 1:1 dimethylacetamide:solutol solution. PBS (112.5 μl) was then slowly added with sonication to obtain a final injection volume of 150 μl. Static and time series images were collected using a customized Olympus FV1000 confocal microscope (Olympus America). A XLUMPLFLN 20 × water immersion objective (NA 1.0) and a 60 × LUMFLN (NA 1.10) water immersion objective were used for data collection (both Olympus America). The imaging drug, H2B-Apple and vascular probes were scanned and excited sequentially using a 405-nm, a 473-nm, a 559-nm and/or a 633-nm diode laser, respectively, in combination with a DM405/488/559/635-nm dichroic beam splitter. Emitted light was then separated and collected using appropriate combinations of beam splitters (SDM473, SDM560 and/or SDM 640) and emission filters BA430-455, BA490-540, BA575-620, BA575-675 and/or BA655-755 (all Olympus America). Control tumours were used to determine settings for voltage and laser power, and to optimize imaging conditions by ensuring that no photobleaching or phototoxicity occurred. Mammary fat pad MDA-MB-231 tumours were grown and imaged as described [50] . MDA-MB-231 cells were injected subcutaneously at the second lowest nipple and grown for 4 weeks. Tumours were exposed for imaging by a medial skin incision. The skin was stretched outward and fixed on a heated cork surface with needles without interfering with blood supply. Image analysis Time-lapse images were analysed using Cell Profiler software [51] . Briefly, cell nuclei were identified by the presence of the fluorescent marker H2B-Apple, which outlined the nucleus. The mean drug signal in the AZD2281-BODIPY FL channel was then measured, and the cell-trafficking function was used to track cells over time. Any overlapping cells were eliminated from the final data set. Histology Five million MDA-MB-231 cells were injected subcutaneously into nude mice and collected after 4 weeks. The tumours were flash-frozen in OCT compound (Sakura Finetek) with isopentane on dry ice, and serial 5-μm thick sections were prepared for immunohistochemistry. Serial sections were stained with PARP-1 (E102: Abcam), PARP-2 (A-18: Santa Cruz Biotechnology, Inc.) and PARP-3 (Sigma-Aldrich) followed by biotinylated secondary antibodies (Vector Laboratories, Inc.). The sections were incubated with 0.3% hydrogen peroxide to block endogenous peroxidase activity, and blocked with 4% normal goat or rabbit serum to reduce non-specific background. ABC kit (Vector Laboratories, Inc.) and AEC substrate (Dako) were used for the colour development, and all the sections were counterstained with Harris haematoxylin (Sigma-Aldrich). The slides were scanned and digitally processed by Nanozoomer 2.0RS (Hamamatsu, Japan). Mathematical model To model drug distribution around tumour blood vessels, a finite element method was implemented using Matlab (Natick, MA). An image of the vascular probe was used to define a two-dimensional layout of microvessels in the field of view. Following automatic mesh generation using a Delaunay triangulation algorithm, the appropriate transport equations and boundary conditions were specified. A mixed (Robin) boundary condition was applied to all vessels, with the plasma concentration set to the experimentally measured biexponential decay. With high-plasma protein binding (>99% bound), the concentration of drug is not depleted along the length of the vessel [29] . The boundary conditions were therefore identical throughout the image. No flux conditions were specified at the image edge. A two-compartment pseudo-homogeneous tissue model was used, where non-specific uptake was assumed to be instantaneous (thereby reducing the effective diffusion coefficient) [52] . Binding to the nuclear target immobilized the drug. Binding and dissociation rates were fit to experimental kinetic rates measured in cell culture and in vitro affinity measurements ( Supplementary Fig. S4 ). Other parameters are listed in Supplementary Fig. S7 . An explicit time-step algorithm was implemented, where the step size was decreased until no overshoot in bound-drug concentration occurred. To visualize the results, a nuclear ‘mask’ was employed where the nuclear concentration was shown within the nuclear region and the non-specific drug concentration was shown outside. This was done for visualization only, as both compartments were simulated in a pseudo-homogeneous tissue. How to cite this article: Thurber, G. M. et al. Single-cell and subcellular pharmacokinetic imaging allows insight into drug action in vivo . Nat. Commun. 4:1504 doi: 10.1038/ncomms2506 (2013).